Combined chemical genetics and data-driven bioinformatics approach identifies receptor tyrosine kinase inhibitors as host-directed antimicrobials Antibiotic resistance poses rapidly increasing global problems in combatting multidrug-resistant (MDR) infectious diseases like MDR tuberculosis, prompting for novel approaches including host-directed therapies (HDT). Intracellular pathogens like Salmonellae and Mycobacterium tuberculosis ( Mtb ) exploit host pathways to survive. Only very few HDT compounds targeting host pathways are currently known. In a library of pharmacologically active compounds (LOPAC)-based drug-repurposing screen, we identify multiple compounds, which target receptor tyrosine kinases (RTKs) and inhibit intracellular Mtb and Salmonellae more potently than currently known HDT compounds. By developing a data-driven in silico model based on confirmed targets from public databases, we successfully predict additional efficacious HDT compounds. These compounds target host RTK signaling and inhibit intracellular (MDR) Mtb . A complementary human kinome siRNA screen independently confirms the role of RTK signaling and kinases (BLK, ABL1, and NTRK1) in host control of Mtb . These approaches validate RTK signaling as a drugable host pathway for HDT against intracellular bacteria. With an estimated 1/4 of the world population carrying a latent Mycobacterium tuberculosis (Mtb) infection, 10.5 million new cases, and 1.8 million deaths annually, tuberculosis (TB) is an increasing global health issue [1] , [2] , [3] . This is further aggravated by the emergence of multi-, extensively, and totally drug-resistant (MDR/XDR/TDR) Mtb strains, threatening to render TB untreatable using current antibiotics [4] , [5] , [6] . In 2015, 480,000 patients suffered from MDR-TB. Although novel candidate antibiotics have recently been identified [7] , current antibiotics already cover the majority of drugable targets of pathogens, resulting in a continuous decline in the number of new and approved antibiotics [8] , [9] , [10] , [11] , [12] , [13] . Intracellular bacteria such as Salmonellae and Mtb pose additional challenges by manipulating host-signaling pathways to subvert innate and adaptive immunity. This, however, also creates potential for novel treatment strategies like host-directed therapy (HDT), to reprogram the host immune system by pharmacological and chemical–genetic manipulation. Importantly, HDT-driven manipulation of host-signaling pathways may be effective also against drug-resistant bacteria, and helps to restore host control of infection in metabolically perturbed cells [14] , [15] . Several recent studies, including our own, have demonstrated the feasibility of HDT approaches to inhibit bacteria both in vitro in human and murine cells [16] , [17] , [18] , [19] , [20] and in vivo in mice, rabbits, and zebrafish [21] , [22] , [23] , [24] , [25] , [26] , [27] , [28] , [29] , [30] , [31] . Using reciprocal chemical genetics targeting the human kinome, we previously identified AKT1 as a central regulator of Salmonella enterica serovar Typhimurium (Stm)- , Mtb- , and MDR- Mtb survival. Treatment of infected cells with the kinase inhibitor H-89 significantly decreased intracellular bacterial loads. Despite H-89 being known as a PKA inhibitor, we demonstrated that this compound inhibited intracellular bacteria by targeting AKT1 [16] . However, H-89 had a substantially lower impact on intracellular growth of Mtb compared to Stm , suggesting that Mtb modulates additional host-signaling pathways to survive. This is in agreement with reports that Mtb arrests vesicle maturation at an earlier stage than Stm [16] , [32] , [33] . Other studies identified additional drugable human kinases that regulate Mtb survival, including TGFβRI and CSNK1 [18] and imatinib-sensitive kinases ABL1 and ABL2 [21] . In addition to kinases and kinase inhibitors, other potential targets and compounds for TB HDT were identified, including two antipsychotics (haloperidol and prochlorperazine) and an antidepressant (nortryptiline) [19] , phosphodiesterase inhibitors [22] , [23] , anti-inflammatory agents like ibuprofen [25] , the FDA-approved drug zileuton [26] , the antidiabetic drug metformin [34] , phenylbutyrate [35] , [36] , and human metabolic targets [37] , [38] . Nevertheless, the field of TB HDT has not fully progressed toward clinical application and many interactions between the host and bacterium remain to be deciphered. Therefore, better compounds are urgently needed as drug candidates for TB HDT, as well as for the identification of cellular events occurring at the host–pathogen interface, which may enable rational drug design for HDT. There are several major challenges to be overcome to facilitate host-directed chemical–genetic studies targeting intracellular pathogens, particularly studies that aim at discovering key host pathways manipulated by Mtb . First, it is extremely difficult to generate sufficient quantities of primary macrophages (Mφs), the natural target cells for Mtb infection, from human donors for medium-throughput screens, even by pheresis. Second, the often-used THP-1 monocytic cell line requires PMA stimulation for differentiation, which massively affects cell signaling and vesicular trafficking [39] , [40] , thus confounding cellular signaling studies. Third, there is a lack of fast (compared to the classical 3-week Mtb colony-forming unit (CFU) assay), robust, and widely applicable readouts for rapid screening. Finally, achieving stable genetic knockdown in human primary macrophages is challenging, especially in large siRNA screens where knockdown efficiency of each individual gene cannot broadly be confirmed. To solve these problems, we have developed a rapid, medium-throughput, fluorescence-based screening assay to determine bacterial load by automated flow cytometry in the highly manipulable human HeLa and MelJuSo cell lines infected with (myco)bacteria expressing novel (myco)bacterial fluorescent protein constructs. Our identification of the MelJuSo cell line as a novel Mtb infection model has several important advantages: MelJuSo cells are suited to large-scale screening assays as they are more homogeneous than primary cells, do not require additional stimuli like PMA for maturation, can be efficiently manipulated using RNAi, and can be infected by mycobacteria [41] . We have shown in the past that human melanocytes can efficiently present mycobacterial antigens to HLA class II-restricted CD4 T cells [42] and have successfully used MelJuSo to dissect molecular pathways of MHC class II presentation in human cells [43] , [44] . Our novel fluorescence-based bacterial growth assay is applicable for both siRNA and chemical compound screens, and is equally suitable for both Stm and Mtb despite the vast differences in their intracellular “lifestyles” and replication rates (20 min and 18 h, respectively) [6] , [32] , [45] , [46] , demonstrating the versatility of this assay. We used this screening assay in drug-repurposing screens, and identified compounds with host-directed anti-(myco)bacterial activity against Mtb and Stm , outperforming published HDT compounds’ activities. Based on these data, together with confirmed target profiles of the screened compounds, we next developed a predictive in silico model in order to be able to identify additional HDT compounds. This model was applied to predict host-directed compounds among all compounds present in the PubChem repository and to identify their key targets with predicted activity against intracellular Stm or Mtb . Interestingly, both our experimental wet lab screens and the novel in silico predictive model identified inhibitors of (growth factor) receptor tyrosine kinases (RTKs) and downstream intermediates of RTK signaling as candidate host-directed drugs to control intracellular infection. Moreover, an siRNA screen of the human kinome in Mtb -infected human cells independently validated a key role for RTK signaling in host control of Mtb . Thus, using two independent chemical–genetic experimental approaches as well as a computational method, we find and validate RTK signaling as a novel important host pathway that controls intracellular Mtb (including MDR- Mtb ) survival. This pathway is druggable by compounds and drugs including clinical drugs such as dovitinib, AT9283, and ENMD-2076. These findings offer new approaches to combat intracellular infectious diseases in the face of rapidly rising multidrug resistance. Flow cytometry-based assay for intracellular bacterial load To allow identification of host-directed drugs and host pathways controlling intracellular bacterial survival, we developed a fast, robust, and novel assay suited for medium-throughput (96-well) compound and siRNA screening. Flow cytometry was used to assay intracellular bacterial load using fluorescent strains of Stm and Mtb . For initial reference purposes, we tested the kinase inhibitor H-89, which we had used in previous work [16] (Supplementary information, Supplementary Figures 1 – 4 ). As mentioned, after screening several cell lines, we identified the MelJuSo cell line as a novel Mtb infection model. To first validate the MelJuSo model system, we tested already-published host-directed compounds with known activity against Mtb here in this model; indeed, as expected, these known compounds also reduced Mtb loads in MelJuSo cells and in human macrophages upon short (overnight) treatment (at standard 10 μM concentrations). 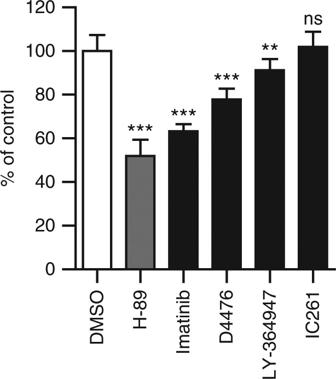Fig. 1 Verification of host-directedMtbinhibitors from literature in the novel screening assay. Overnight treatment of MelJuSo cells infected withMtbconstitutively expressing stable DsRed with compounds that were previously reported to be active againstMtbat 10 µM or with DMSO at equal v/v. H-89 is used as a positive control at 10 µM16. TheMtbbacterial load is displayed as a percentage of the DMSO control ± standard deviation to indicate the extent of bacterial inhibition. Statistically significant difference compared to DMSO was tested using a one-way ANOVA. (ns not significant, **pvalue < 0.01, ***pvalue < 0.001) Supplementary Figure 1 describes the assay in more detail. As shown in Fig. 1 , imatinib, D4476, and LY-364947 all decreased the Mtb bacterial load in our model, which was well in agreement with previous studies [18] , [21] . In addition, we also confirmed that a dual inhibitor of TGFbetaR1 and casein kinase 1 (D4476) inhibited Mtb more potently than the individual inhibitors of TGFbetaR1 (LY-364947) and casein kinase 1 (IC261) alone, confirming data from Jayaswal et al. [18] (Fig. 1 ). Finally, during the work described in this paper also, haloperidol [19] was confirmed to inhibit both Stm and Mtb in our model (Table 1 ) and these results will be discussed in more detail below. Thus, the results obtained in our novel MelJuSo- Mtb infection model and flow cytometry-based readout of intracellular infection faithfully reproduce the reported inhibitory effects of previously published compounds, providing important biological plausibility for the system. Fig. 1 Verification of host-directed Mtb inhibitors from literature in the novel screening assay. Overnight treatment of MelJuSo cells infected with Mtb constitutively expressing stable DsRed with compounds that were previously reported to be active against Mtb at 10 µM or with DMSO at equal v/v. H-89 is used as a positive control at 10 µM [16] . The Mtb bacterial load is displayed as a percentage of the DMSO control ± standard deviation to indicate the extent of bacterial inhibition. Statistically significant difference compared to DMSO was tested using a one-way ANOVA. (ns not significant, ** p value < 0.01, *** p value < 0.001) Full size image Table 1 Details of validated hit compounds from the Mtb and Stm LOPAC screens Full size table Of note, none of the published compounds evaluated above was more potent in inhibiting intracellular Mtb than our reference compound H-89. We therefore used our assay to screen chemical libraries to identify host-directed inhibitors with more potent activity than H-89. Identification of host-directed antimicrobial compounds We next applied the novel screening assay for a TB drug-repurposing screen of a library of 1260 pharmacologically active compounds (LOPAC) in order to identify host-directed compounds with stronger activity against intracellular Mtb than H-89. The primary screen in the MelJuSo- Mtb intracellular infection model identified 110 compounds that significantly reduced and 16 compounds that increased intracellular bacterial loads. Ninety of these did not affect host cell viability (Fig. 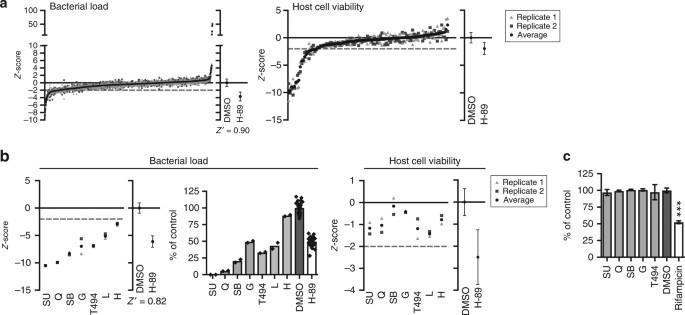Fig. 2 Identification of host-directed compounds inhibitingMtb.aResults of a screen of 1260 compounds of the LOPAC library at 10 µM in the MelJuSo-Mtbinfection model usingMtbconstitutively expressing stable DsRed, expressed asz-scores (left panel). Individual replicates of the screened compounds are shown as gray points and the averagez-score for each compound is displayed in black. The averagez-score and standard deviation of the controls (DMSO and H-89) are displayed separately and the assay window expressed as a Z′-factor is shown below. Cell viabilityz-scores of the 110 hit compounds are shown in the right panel. The dashed line depicts a cutoff at az-score of −2.bA rescreen of the hit compounds that were superior to H-89 without affecting cell viability at 10 µM is shown as ina. The bacterial load is expressed as az-score in the utmost left panel and as a percentage of control value in the middle panel to indicate the extent of bacterial inhibition. Individual screening datapoints are overlayed on the bar graph. Compound abbreviations: SU = SU 6656, Q = quinacrine, SB = SB 216763, G = GW5074, T494 = tyrphostin AG 494, L = L-594,881, H = haloperidol.cMtbbroth culture treated for 6 days with the five hit compounds of theMtbscreen at 10 µM. Rifampicin (20 μg/ml) was used as a positive control. The average bacterial density ± standard deviation of four replicates from a representative experiment (out of three experiments) is shown, expressed as a percentage of the DMSO control. Statistically significant difference compared to DMSO was tested using a one-way ANOVA (F(6,25)= 81.66; ***pvalue < 0.001) 2a and Supplementary Table 2 ) and were therefore pursued further. Seven compounds decreased Mtb bacterial load more potently than H-89 (Table 1 ). A rescreen of these seven compounds confirmed their activity and five of these compounds again surpassed H-89 (SU 6656, quinacrine, SB 216763, GW5074, and tyrphostin AG 494; Fig. 2b and Table 1 ). Figure 2b shows z -score values in the left panel, with the actual percentage inhibition of Mtb growth shown in the middle panel, expressed as the % of control value. These latter data confirmed the strong inhibitory effect of these HDT compounds on intracellular Mtb . We next confirmed that these compounds exerted their antimicrobial effects via the host by excluding any direct microbicidal activity against extracellular Mtb (Fig. 2c ). As a control, the classical Mtb antibiotic rifampicin significantly inhibited Mtb . Fig. 2 Identification of host-directed compounds inhibiting Mtb . a Results of a screen of 1260 compounds of the LOPAC library at 10 µM in the MelJuSo- Mtb infection model using Mtb constitutively expressing stable DsRed, expressed as z -scores (left panel). Individual replicates of the screened compounds are shown as gray points and the average z -score for each compound is displayed in black. The average z -score and standard deviation of the controls (DMSO and H-89) are displayed separately and the assay window expressed as a Z′-factor is shown below. Cell viability z -scores of the 110 hit compounds are shown in the right panel. The dashed line depicts a cutoff at a z -score of −2. b A rescreen of the hit compounds that were superior to H-89 without affecting cell viability at 10 µM is shown as in a . The bacterial load is expressed as a z -score in the utmost left panel and as a percentage of control value in the middle panel to indicate the extent of bacterial inhibition. Individual screening datapoints are overlayed on the bar graph. Compound abbreviations: SU = SU 6656, Q = quinacrine, SB = SB 216763, G = GW5074, T494 = tyrphostin AG 494, L = L-594,881, H = haloperidol. c Mtb broth culture treated for 6 days with the five hit compounds of the Mtb screen at 10 µM. Rifampicin (20 μg/ml) was used as a positive control. The average bacterial density ± standard deviation of four replicates from a representative experiment (out of three experiments) is shown, expressed as a percentage of the DMSO control. Statistically significant difference compared to DMSO was tested using a one-way ANOVA (F (6,25) = 81.66; *** p value < 0.001) Full size image To investigate whether compounds also existed with host-directed activity against Stm , and whether their activity was selective for Mtb , Stm, or both, we also screened the same LOPAC library using the very similar HeLa- Stm infection model (Fig. 3a ). 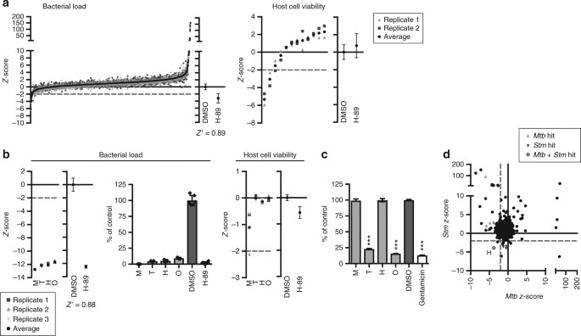Fig. 3 Identification of host-directed compounds inhibitingStm.aScreen of the LOPAC library in the HeLa-Stminfection model usingStmconstitutively expressing stable DsRed, as in Fig.2a.bRescreen of the hit compounds from the HeLa-Stmscreen that were superior to H-89 without affecting cell viability, displayed as in Fig.2b. The bacterial load is expressed as az-score in the utmost left panel and as a percentage of control value ± standard deviation in the middle panel to indicate the extent of bacterial inhibition. Compound abbreviations: T = trimethoprim, H = haloperidol, M = mibefradil, O = ofloxacin.cOvernight treatment of aStmbroth culture with the hit compounds at 10 µM. Gentamicin (50 μg/ml) was used as a positive control. The average bacterial density ± standard deviation of six replicates from a representative experiment out of three experiments is shown. The bacterial load is expressed as a percentage of the DMSO control value to indicate the extent of bacterial inhibition. Statistically significant difference compared to DMSO was tested using a one-way ANOVA (F(5,30)= 4871; ***pvalue < 0.001).dComparison of theStmandMtbprimary screening data. Compounds that were superior to H-89 and subsequently confirmed in a rescreen are indicated in gray triangles. H = haloperidol Twelve compounds were identified that significantly reduced the Stm bacterial load and 10 of these did not affect host cell viability (Supplementary Table 3 ). A total of 173 compounds increased the Stm bacterial load without affecting host cell viability. Four of the hit compounds that decreased the bacterial load (trimethoprim, haloperidol, mibefradil, and ofloxacin) were superior to H-89 in inhibiting intracellular Stm (Table 1 ). Mibefradil again exceeded the inhibitory effect of H-89 in a rescreen (Fig. 3b ), while all four compounds consistently and strongly decreased the Stm bacterial load. While Fig. 3a and the left panel of Fig. 3b show z -score values, the percentage inhibition of intracellular Stm growth is shown in the middle panel of Fig. 3b , expressed as the % of control value, demonstrating the strong inhibitory effect of these HDT compounds on intracellular Stm . We next excluded any direct microbicidal activity of these HDT compounds against extracellular Stm (Fig. 3c ). By contrast, trimethoprim and ofloxacin (both known antibiotics), which were part of the LOPAC library and therefore tested here as well, directly inhibited extracellular Stm as expected. The fact that these known antibiotics for Stm were hits in our screen further confirms the strength and validity of our approach, showing that we can clearly distinguish antibiotics from host-directed compounds. Taken together, haloperidol (a known HDT inhibitor [19] ) and mibefradil (newly discovered here) were confirmed and identified, respectively, as host-directed inhibitors of Stm . Fig. 3 Identification of host-directed compounds inhibiting Stm . a Screen of the LOPAC library in the HeLa- Stm infection model using Stm constitutively expressing stable DsRed, as in Fig. 2a . b Rescreen of the hit compounds from the HeLa- Stm screen that were superior to H-89 without affecting cell viability, displayed as in Fig. 2b . The bacterial load is expressed as a z -score in the utmost left panel and as a percentage of control value ± standard deviation in the middle panel to indicate the extent of bacterial inhibition. Compound abbreviations: T = trimethoprim, H = haloperidol, M = mibefradil, O = ofloxacin. c Overnight treatment of a Stm broth culture with the hit compounds at 10 µM. Gentamicin (50 μg/ml) was used as a positive control. The average bacterial density ± standard deviation of six replicates from a representative experiment out of three experiments is shown. The bacterial load is expressed as a percentage of the DMSO control value to indicate the extent of bacterial inhibition. Statistically significant difference compared to DMSO was tested using a one-way ANOVA (F (5,30) = 4871; *** p value < 0.001). d Comparison of the Stm and Mtb primary screening data. Compounds that were superior to H-89 and subsequently confirmed in a rescreen are indicated in gray triangles. H = haloperidol Full size image Interestingly, a comparison of the Mtb and Stm HDT compound screening results revealed a highly limited overlap between hits in the two infection models (Fig. 3d ). This observation agrees well with reports that Mtb and Stm arrest vesicle maturation at different stages [16] , [32] , [33] . Haloperidol was the only compound that inhibited both Mtb and Stm . Identification of HDT compounds using an in silico model We next decided to use the above experimental data obtained in our LOPAC screens, and combine these with bioactivity assay-based data available for all 1260 LOPAC compounds in PubChem, to develop a novel bioinformatics predictive model using machine learning. The model was constructed to predict new chemical compounds with host-directed activity against intracellular Stm or Mtb , based on target protein profiles identified by machine learning from our own LOPAC screening data (Fig. 4a ). In the Supplementary Information, an extended description of the machine-learning methods is provided describing the predictive model. In brief, we first linked all LOPAC compounds to PubChem, and retrieved bioassay data by using a preprocessing pipeline (Supplementary Figure 5a ), which identified 1058 confirmed human protein targets for these 1260 compounds. 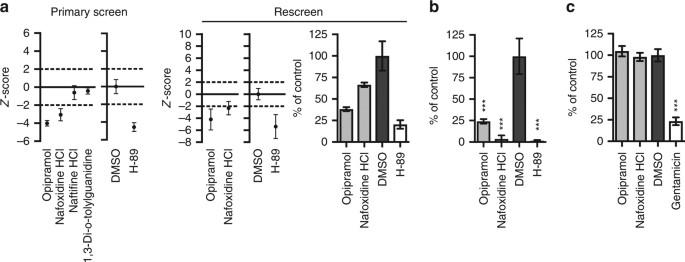Fig. 5 Screen of in silico-predicted chemical compounds active against intracellularStm.aChemical compound primary screen (left panel) and rescreen (middle panel) at 10 µM in the HeLa-Stminfection model usingStmconstitutively expressing stable DsRed, expressed as meanz-scores ± standard deviation. Horizontal dashed lines indicate a hit cutoff at az-score of 2 or −2. The averagez-scores and standard deviations of the controls (DMSO and H-89) are displayed separately. To indicate the extent of bacterial inhibition, rescreen results are expressed as a percentage of control value ± standard deviation in the right panel.bCFU assay of the HeLa-Stminfection model treated with the validated hit compounds fromaat 10 µM. Representative data out of three independent experiments, displayed as a percentage of the DMSO control are shown. The average ± standard deviation of three replicates is shown. Statistically significant differences compared to DMSO were tested using a one-way ANOVA (F(3,8)= 56.31; ***pvalue < 0.001).cOvernight treatment ofStmbroth cultures with the hit compounds at 10 µM. TheStmantibiotic gentamicin (50 μg/ml) was used as a positive control. The average bacterial density ± standard deviation of three replicates is shown, expressed as a percentage of the DMSO control. Representative results out of three individual experiments are displayed. Statistically significant differences compared to DMSO were tested using a one-way ANOVA (F(3,38)= 579.5; ***pvalue < 0.001) 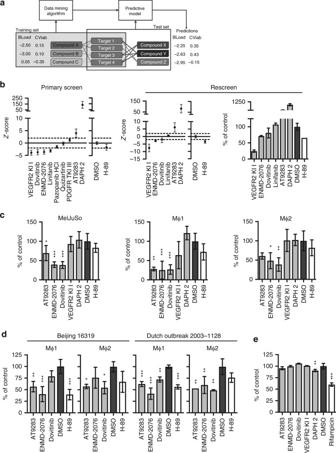This resulted in a data table comprising all LOPAC compounds annotated with their corresponding impact on intracellular bacterial survival and host cell viability from our screens, expressed as z -scores, and combined with their PubChem bioassay activity for each confirmed human target. Fig. 4 Screen of in silico-predicted chemical compounds active against intracellularMtb.aSchematic overview of the in silico predictive model. BLoad = bacterial loadz-score, CViab = cell viabilityz-score.bChemical compound primary screen (left panel) and rescreen (middle panel) at 10 µM in the MelJuSo-Mtbinfection model usingMtbconstitutively expressing stable DsRed, expressed as meanz-scores ± standard deviation. Horizontal dashed lines indicate a hit cutoff at az-score of 2 or −2. The averagez-score and standard deviation of the controls (DMSO and H-89) are displayed separately. To indicate the extent of bacterial inhibition, rescreen results are expressed both asz-score and as a percentage of control value ± standard deviation in the right panel.cCFU assay of the MelJuSo (left panel) and human primary Mφ1 (middle panel) and Mφ2 (right panel)Mtbinfection models treated with the validated hit compounds frombat 10 µM. Mφ1 and Mφ2 models have been described by Verreck et al.78. Representative data out of three independent experiments (MelJuSo) and data from a representative donor (Mφs) out of two (Mφ1) or five (Mφ2) different healthy blood bank donors are shown. To indicate the extent of bacterial inhibition, the results are expressed as a percentage of control value ± standard deviation. Number of replicates in the MelJuSo model: AT9283 and ENMD-2076:n= 6; dovitinib, VEGFR KI I, and DAPH 2:n= 5; DMSO and H-89:n= 9. Number of replicates in the Mφ models: AT9283, ENMD-2076, dovitinib, VEGFR KI I, and DAPH 2:n= 3; DMSO and H-89:n= 5. Statistically significant difference compared to DMSO was tested using a one-way ANOVA (MelJuSo: F(6,39)= 16.35; Mφ1: F(6,18)= 10.88; Mφ2: F(6,18)= 5.23; *pvalue < 0.05, **pvalue < 0.01, ***pvalue < 0.001).dCFU assay of the human primary Mφ1 and Mφ2 models infected with two different MDR-Mtbstrains (Beijing family China 16319 and Dutch outbreak 2003-1128) and treated with the validated hit compounds fromcat 10 µM. Data (n= 3 technical replicates) from a representative donor out of four different healthy blood bank donors, displayed as a percentage of the DMSO control ± standard deviation are shown. Statistically significant differences compared to DMSO were tested using a one-way ANOVA (Mφ1 Beijing: F(4,10)= 11.43; Mφ2 Beijing: F(4,10)= 3.72; Mφ1 Dutch outbreak: F(4,10)= 29.09; Mφ2 Dutch outbreak: F(4,10)= 8.81; *pvalue < 0.05, **pvalue < 0.01, ***pvalue < 0.001).eSix-day treatment ofMtbbroth cultures with the hit compounds at 10 µM. TheMtbantibiotic rifampicin (20 μg/ml) was used as a positive control. The average bacterial density ± standard deviation of three replicates is shown, expressed as a percentage of the DMSO control. Representative results out of three individual experiments are displayed. Statistically significant difference compared to DMSO was tested using a one-way ANOVA (F(6,25)= 101.4; **pvalue < 0.01, ***pvalue < 0.001) An example of the table structure is shown in Supplementary Table 4 . This was then used as a training set to learn ensembles of predictive clustering trees (PCTs; Supplementary Figure 5c ) to predict the impact on intracellular bacterial survival and host cell viability. We next employed this in silico tool (the learned model) to identify and select candidate compounds from PubChem with predicted host-directed antimicrobial activity. Querying PubChem for compounds that are known to target one or more of the above 1058 confirmed human protein targets yielded 460,580 compounds, which were then annotated with their bioassay data and fed into the predictive model as a testing set. 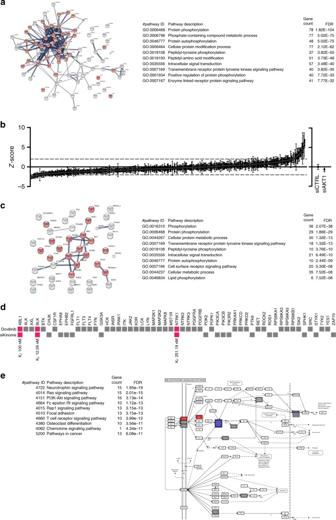Fig. 6 Identification of host kinases controlling intracellularMtbsurvival.aSTRING network of confirmed targets of dovitinib retrieved from the ChEMBL repository Compound Bioactivity section (left panel). Individual proteins are displayed as nodes. Lines represent protein–protein interactions and the thickness of the lines indicates confidence. Proteins participating in the “transmembrane receptor tyrosine kinase signaling pathway” are displayed in red. The top 10 enriched GO terms in the “Biological Function” category are displayed along with the number of genes/proteins annotated with the indicated GO terms and the false-discovery rate (FDR) of the enrichment (right panel).bResults of a siRNA screen of the human kinome in the MelJuSo-Mtbinfection model usingMtbconstitutively expressing destabilized DsRed, expressed asz-scores. The averagez-score ± standard deviation for each siRNA pool is displayed. A hit cutoff atz= 2 orz= –2 is displayed as a dashed line. The averagez-score and standard deviation of the controls (siCTRL and siAKT) are displayed separately. SiCTRL: nontargeting siRNA pool.cSTRING network of the siRNA screen hits (left panel) is displayed along the top 10 enriched GO terms in the “Biological Function” category (right panel), as ina.dParticipation of individual targets of dovitinib (top row) or hits from the siRNA screen (bottom row) in the “transmembrane receptor tyrosine kinase signaling pathway” are indicated by filled squares. Proteins that are both targeted by dovitinib and were a hit in the siRNA screen are shown in magenta. Dissociation constants (Ki) retrieved from ChEMBL are shown below for the interaction between dovitinib and ABL1, BLK, and NTRK1.eSTRING analysis to identify enriched KEGG pathways using the kinases fromd. The top 10 enriched KEGG pathways along with the number of genes/proteins annotated with the indicated GO terms and the FDR of the enrichment are displayed (left panel). Involvement of individual proteins is overlaid on the “neurotrophin signaling pathway” KEGG pathway retrieved from the Kyoto Encyclopedia of Genes and Genomes (http://www.genome.jp/kegg/). Proteins in gray are targeted by dovitinib only, blue proteins were siRNA screening hits, and proteins in red are both targeted by dovitinib and silencing of these genes affected theMtbbacterial load Using the ensembles of PCTs learned from the training data to predict the intracellular bacterial survival and host cell viability z -scores of these 460,580 compounds, we identified 47 candidate compounds predicted to affect intracellular Mtb load (Supplementary Table 5 ) and 30 compounds predicted to affect intracellular Stm load (Supplementary Table 6 ). From these two lists of compounds, commercially available compounds (Table 2 ) were ordered and screened in the MelJuSo- Mtb and HeLa- Stm infection models. As the PubChem BioAssay data contain compound–target relations based only on IC 50 and EC 50 values as well as binding constants, the predictive model was able to identify only compound–target interactions rather than the direction of the target effects. Thus, as we were therefore unable to predict whether compounds would actually inhibit or activate their associated targets, predicted negative z -scores might result in experimentally positive z -scores in in vitro intracellular bacterial inhibition tests and vice versa. In the Mtb screen, six out of nine compounds predicted to affect the bacterial load indeed decreased or increased the bacterial load (Fig. 4b , left panel). A rescreen of the hit compounds confirmed five out of six hits (VEGFR KI I, ENMD-2076, dovitinib, AT9283, and DAPH 2; Fig. 4b , middle and right panels). The results are shown as z -scores as well as the percentage inhibition of Mtb growth expressed as the % of control value, to confirm the strong inhibitory effect of these HDT compounds on intracellular Mtb (Fig. 4b , outer right panel). Fig. 4 Screen of in silico-predicted chemical compounds active against intracellular Mtb . a Schematic overview of the in silico predictive model. BLoad = bacterial load z -score, CViab = cell viability z -score. b Chemical compound primary screen (left panel) and rescreen (middle panel) at 10 µM in the MelJuSo- Mtb infection model using Mtb constitutively expressing stable DsRed, expressed as mean z -scores ± standard deviation. Horizontal dashed lines indicate a hit cutoff at a z -score of 2 or −2. The average z -score and standard deviation of the controls (DMSO and H-89) are displayed separately. To indicate the extent of bacterial inhibition, rescreen results are expressed both as z -score and as a percentage of control value ± standard deviation in the right panel. c CFU assay of the MelJuSo (left panel) and human primary Mφ1 (middle panel) and Mφ2 (right panel) Mtb infection models treated with the validated hit compounds from b at 10 µM. Mφ1 and Mφ2 models have been described by Verreck et al. [78] . Representative data out of three independent experiments (MelJuSo) and data from a representative donor (Mφs) out of two (Mφ1) or five (Mφ2) different healthy blood bank donors are shown. To indicate the extent of bacterial inhibition, the results are expressed as a percentage of control value ± standard deviation. Number of replicates in the MelJuSo model: AT9283 and ENMD-2076: n = 6; dovitinib, VEGFR KI I, and DAPH 2: n = 5; DMSO and H-89: n = 9. Number of replicates in the Mφ models: AT9283, ENMD-2076, dovitinib, VEGFR KI I, and DAPH 2: n = 3; DMSO and H-89: n = 5. Statistically significant difference compared to DMSO was tested using a one-way ANOVA (MelJuSo: F (6,39) = 16.35; Mφ1: F (6,18) = 10.88; Mφ2: F (6,18) = 5.23; * p value < 0.05, ** p value < 0.01, *** p value < 0.001). d CFU assay of the human primary Mφ1 and Mφ2 models infected with two different MDR- Mtb strains (Beijing family China 16319 and Dutch outbreak 2003-1128) and treated with the validated hit compounds from c at 10 µM. Data ( n = 3 technical replicates) from a representative donor out of four different healthy blood bank donors, displayed as a percentage of the DMSO control ± standard deviation are shown. Statistically significant differences compared to DMSO were tested using a one-way ANOVA (Mφ1 Beijing: F (4,10) = 11.43; Mφ2 Beijing: F (4,10) = 3.72; Mφ1 Dutch outbreak: F (4,10) = 29.09; Mφ2 Dutch outbreak: F (4,10) = 8.81; * p value < 0.05, ** p value < 0.01, *** p value < 0.001). e Six-day treatment of Mtb broth cultures with the hit compounds at 10 µM. The Mtb antibiotic rifampicin (20 μg/ml) was used as a positive control. The average bacterial density ± standard deviation of three replicates is shown, expressed as a percentage of the DMSO control. Representative results out of three individual experiments are displayed. Statistically significant difference compared to DMSO was tested using a one-way ANOVA (F (6,25) = 101.4; ** p value < 0.01, *** p value < 0.001) Full size image Table 2 Compounds selected from the predictive model output Full size table As compound autofluorescence might result in false-positive z -scores in our assay, we further validated all the confirmed hit compounds independently in classical CFU assays, both in cell lines and in primary human macrophages. The compounds AT9283, ENMD-2076, and dovitinib significantly decreased Mtb CFUs in both MelJuSo cells and human primary Mφs (Fig. 4c ; results are shown as percentage inhibition of Mtb growth expressed as % of control value). Importantly, AT9283, ENMD-2076, and dovitinib also reduced CFUs in human primary macrophages infected with two different MDR- Mtb strains (Beijing family China 16319 and Dutch outbreak 2003-1128; Fig. 4d ). These data independently confirm and validate the results obtained in our novel screening and prediction pipeline, and importantly extend the newly identified HDT compounds’ effects to intracellular multidrug-resistant bacteria. Finally, none of the compounds directly affected extracellular bacterial growth in liquid cultures, while classical antibiotics (rifampicin) did, confirming that the mode of action of the new HDT compounds is via modulation of host and not direct bacterial mechanisms (Fig. 4e ). Using this same screening and validation approach for Stm in the HeLa- Stm infection model, we confirmed that two out of four compounds predicted to affect Stm survival indeed decreased the bacterial load of Stm -infected cells in a primary screen (Fig. 5a , left panel). Both of these hits (opipramol and nafoxidine) were subsequently confirmed in a rescreen (Fig. 5a , middle and right panels; results shown as z -scores and as % inhibition of Stm growth expressed as the % of control value). Both hit compounds also reduced the Stm bacterial load independently in classical CFU assays (Fig. 5b ), again without directly affecting bacterial growth in a liquid overnight Stm culture (Fig. 5c ), confirming their HDT mode of action. These data therefore confirm and validate our novel screening and prediction pipeline not only for Mtb , but also for Stm . Fig. 5 Screen of in silico-predicted chemical compounds active against intracellular Stm . a Chemical compound primary screen (left panel) and rescreen (middle panel) at 10 µM in the HeLa- Stm infection model using Stm constitutively expressing stable DsRed, expressed as mean z -scores ± standard deviation. Horizontal dashed lines indicate a hit cutoff at a z -score of 2 or −2. The average z -scores and standard deviations of the controls (DMSO and H-89) are displayed separately. To indicate the extent of bacterial inhibition, rescreen results are expressed as a percentage of control value ± standard deviation in the right panel. b CFU assay of the HeLa- Stm infection model treated with the validated hit compounds from a at 10 µM. Representative data out of three independent experiments, displayed as a percentage of the DMSO control are shown. The average ± standard deviation of three replicates is shown. Statistically significant differences compared to DMSO were tested using a one-way ANOVA (F (3,8) = 56.31; *** p value < 0.001). c Overnight treatment of Stm broth cultures with the hit compounds at 10 µM. The Stm antibiotic gentamicin (50 μg/ml) was used as a positive control. The average bacterial density ± standard deviation of three replicates is shown, expressed as a percentage of the DMSO control. Representative results out of three individual experiments are displayed. Statistically significant differences compared to DMSO were tested using a one-way ANOVA (F (3,38) = 579.5; *** p value < 0.001) Full size image Thus, we have successfully developed and used a data-driven novel in silico predictive model to identify host-directed compounds with antimicrobial activity against intracellular bacteria. The model significantly enhanced the identification of de novo hit compounds (5 out of 9 (55.6%) and 2 out of 4 (50%) for Mtb and Stm , respectively) compared to random LOPAC library primary screening (126 out of 1260 (10%) for Mtb and 185 out of 1260 (14.6%) for Stm ). In addition, the results were replicated and validated in primary human Mφs infected with Mtb , strongly agreeing with and further validating the MelJuSo- Mtb model used in our novel flow cytometry-based screening assay. RTK signaling is a novel host pathway controlling Mtb As AT9283, ENMD-2076, and dovitinib are RTK inhibitors [47] , [48] , [49] , we used a chemical genetics approach to confirm a role for RTK signaling in host-mediated Mtb control. We first retrieved human protein targets of AT9283, ENMD-2076, and dovitinib from the Compound Bioactivity section in ChEMBL ( http://www.www.ebi.ac.uk/chembl/ ) and further downselected targets for which the compounds were annotated as “Active.” Because no targets annotated as “Active” could be retrieved for AT9283 and ENMD-2076, we first constructed a STRING protein network and performed gene ontology (GO) analysis using the targets of dovitinib ( n = 86 proteins; Fig. 6a ). Due to the hierarchical organization of GO terms, general cellular and molecular functions tend to be highly enriched in GO term enrichment analyses. Therefore, we focused on identifying the highest-ranked GO terms that described distinct pathways rather than the overall highest-ranked GO terms. As expected from the reported target specificities of dovitinib [49] , “transmembrane receptor protein tyrosine kinase signaling pathway” (GO:0007169, false-discovery rate (FDR) 3.82E−33) was the highest-ranking enriched pathway and 40 protein targets participated in this pathway (Fig. 6a and Supplementary Figure 6a ). We next verified that both AT9283 and ENMD-2076 target RTKs by retrieving human protein targets from the Target Summary section in ChEMBL and performed an identical STRING analysis (Supplementary Figure 6b, c ). Even though this analysis resulted in small networks due to the limited number of studied targets and the lists of targets from the Target Summary section also include nonconfirmed targets, the GO term “transmembrane receptor protein tyrosine kinase signaling pathway” (GO:0007169) was again highly enriched in the target networks of AT9283 (FDR 1.11E−12) and ENMD-2076 (FDR 6.47E−5). Fig. 6 Identification of host kinases controlling intracellular Mtb survival. a STRING network of confirmed targets of dovitinib retrieved from the ChEMBL repository Compound Bioactivity section (left panel). Individual proteins are displayed as nodes. Lines represent protein–protein interactions and the thickness of the lines indicates confidence. Proteins participating in the “transmembrane receptor tyrosine kinase signaling pathway” are displayed in red. The top 10 enriched GO terms in the “Biological Function” category are displayed along with the number of genes/proteins annotated with the indicated GO terms and the false-discovery rate (FDR) of the enrichment (right panel). b Results of a siRNA screen of the human kinome in the MelJuSo- Mtb infection model using Mtb constitutively expressing destabilized DsRed, expressed as z -scores. The average z -score ± standard deviation for each siRNA pool is displayed. A hit cutoff at z = 2 or z = –2 is displayed as a dashed line. The average z -score and standard deviation of the controls (siCTRL and siAKT) are displayed separately. SiCTRL: nontargeting siRNA pool. c STRING network of the siRNA screen hits (left panel) is displayed along the top 10 enriched GO terms in the “Biological Function” category (right panel), as in a . d Participation of individual targets of dovitinib (top row) or hits from the siRNA screen (bottom row) in the “transmembrane receptor tyrosine kinase signaling pathway” are indicated by filled squares. Proteins that are both targeted by dovitinib and were a hit in the siRNA screen are shown in magenta. Dissociation constants ( K i ) retrieved from ChEMBL are shown below for the interaction between dovitinib and ABL1, BLK, and NTRK1. e STRING analysis to identify enriched KEGG pathways using the kinases from d . The top 10 enriched KEGG pathways along with the number of genes/proteins annotated with the indicated GO terms and the FDR of the enrichment are displayed (left panel). Involvement of individual proteins is overlaid on the “neurotrophin signaling pathway” KEGG pathway retrieved from the Kyoto Encyclopedia of Genes and Genomes ( http://www.genome.jp/kegg/ ). Proteins in gray are targeted by dovitinib only, blue proteins were siRNA screening hits, and proteins in red are both targeted by dovitinib and silencing of these genes affected the Mtb bacterial load Full size image To independently confirm RTK signaling as a functional pathway that controls intracellular survival of Mtb , we next performed an unbiased siRNA screen of the human kinome in the MelJuSo- Mtb infection model (Fig. 6b ), agnostic to the above data. The siRNA screen identified 20 targets that decreased and 21 that increased the Mtb bacterial load while not affecting host cell viability (Table 3 ). These 41 hit kinases were then used in a STRING protein network and GO analysis. Independently confirming the STRING analysis of the targets of dovitinib, AT9283, and ENMD-2076, also, in this analysis, again “transmembrane receptor protein tyrosine kinase signaling pathway” (GO:0007169, FDR 1.32E−13) was the highest-ranking enriched pathway, and 18 hit kinases from the siRNA screen participated in this pathway (Fig. 6c and Supplementary Figure 6d ). Three of the kinases (ABL1, BLK, and NTRK1) were both hits in the siRNA screen and confirmed targets of dovitinib (Fig. 6d ). Of these three kinases, only ABL1 was present in the potential target networks of AT9283 and ENMD-2076 (Supplementary Figure 6 b, c). However, a lower dissociation constant ( K i ) is reported in ChEMBL for the interaction between dovitinib and BLK ( K i : 12.59 nM) than between dovitinib and ABL1 ( K i : 100 nM), suggesting that BLK is targeted more strongly by dovitinib. To identify the top-enriched RTK signaling pathway targeted by dovitinib and siRNA, we used the kinases shown in Fig. 6d in a STRING analysis. This identified the neurotrophin signaling pathway as the top-enriched KEGG pathway (Fig. 6e ) [50] . Silencing of neurotrophic receptor tyrosine kinase 1 (NTRK1) resulted in an increased Mtb bacterial load (Table 3 ), establishing a functional link between neurotrophin signaling and Mtb survival. Table 3 siKinome screen hits in the MelJuSo- Mtb infection model Full size table Thus, using independent chemical, genetic, functional, and computational approaches, we find and validate that (1) RTK signaling is a novel host pathway that controls intracellular (MDR)- Mtb survival and that (2) repurposable drugs such as dovitinib, AT9283, and ENMD-2076 that target RTK signaling are new candidates for HDT in treating TB, including multidrug-resistant Mtb . Employing chemical genetic screens complemented with newly developed computational approaches, we have identified host-directed therapy (HDT) compounds and drugs (dovitinib, AT9283, and ENMD-2076) that target human RTK signaling to control intracellular Mtb survival, including MDR- Mtb . Perhaps, more importantly, our findings pave the way toward identifying additional compounds targeting human RTK signaling to improve control of intracellular Mtb infection since all compounds were confirmed to be effective in primary human macrophage infection models. Current efforts to develop HDT are a topic of interest for infectious diseases and cancer (reviewed recently [38] ). In order to be able to screen larger HDT compound libraries for novel leads with activity against intracellular Mtb and Stm , we have developed a new robust and rapid fluorescence-based intracellular screening assay. This assay allowed us to identify host-directed Mtb -inhibiting compounds (SU 6656, quinacrine, SB 216763, GW5074, and tyrphostin AG 494) and host-directed Stm -inhibiting compounds (mibefradil), which performed significantly better than our best reference compound H-89, in a LOPAC library drug-repurposing screening effort. We were also able to confirm the activity of previously published HDT compounds in our screening approach (imatinib, D4476, LY-364947, and haloperidol), lending strong plausibility and validity to our strategy. We next developed a novel in silico model which was data driven and based on known and confirmed targets from public databases, by which we could successfully predict and verify additional compounds with host-directed activity against Mtb (dovitinib, AT9283, and ENMD-2076) and Stm (nafoxidine and opipramol). Using STRING network analysis, we uncovered RTK signaling as a novel host pathway controlling Mtb intracellular survival, which is targeted by compounds identified in this study. Finally, we performed an independent unbiased siRNA screen of the human kinome, which confirmed a role for RTK signaling in control of intracellular Mtb survival. Collectively, our results uncover new host-signaling pathways as well as the corresponding active chemical compounds targeting these to control intracellular bacterial infections, including MDR-TB and Stm . Our LOPAC screen provides an important and general proof of principle for drug repurposing, since we successfully identified several candidate compounds that displayed host-directed antimicrobial activity while their known targets have not previously been associated with infectious diseases. Strikingly, four of the five hit compounds that consistently outperformed H-89 in controlling Mtb infection are known to affect (growth factor) RTK signaling. Tyrphostin AG 494, SU 6656, SB 216763, and GW5074 are inhibitors of EGFR, SRC family kinases (SFKs), GSK-3, and RAF1, respectively, which are all kinases participating in RTK pathways [51] , [52] , [53] , [54] , [55] . In addition to compounds affecting RTK signaling, we identified three other host-directed Mtb -inhibiting compounds with vastly different target specificities. First, quinacrine was originally developed as an antimalarial drug but has displayed activity in a myriad of diseases via a wide range of targets [56] . Interestingly, reported targets of quinacrine include AKT1 and NF-κB as well as phospholipase A2 [57] . The latter is a central enzyme in the eicosanoid pathway, which was recently shown to be involved in Mtb control by balancing the type I interferon response [26] . Second, haloperidol is an antipsychotic drug targeting dopamine receptors [58] . Importantly, haloperidol was recently shown to affect survival of intracellular mycobacteria in a host-directed fashion [19] , providing important additional and independent validation of our screening strategy and models. Finally, 3′,4′-dichlorobenzamil is an amiloride-analog Na + /Ca 2+ exchanger inhibitor [59] . This compound may act by inhibiting Ca 2+ transport in the cell, as activation of calcineurin by increased Ca 2+ levels has previously been proposed as a mechanism for inhibition of phagosome maturation in Mtb -infected cells [60] . A similar LOPAC library screen in the HeLa- Stm infection model resulted in four compounds that more strongly reduced the bacterial load than our reference compound H-89, and mibefradil was further confirmed to surpass H-89’s activity in a rescreen. However, H-89 is already a highly potent host-directed inhibitor of Stm and all four compounds consistently and significantly reduced the Stm bacterial load. Two of the four hit compounds from the primary screen were known antibiotics (trimethoprim and ofloxacin) but these were tested nevertheless in our screen because they were part of the LOPAC. Of the remaining two HDT compounds, haloperidol, which was already found in a previous HDT screen study in TB, was confirmed as a HDT compound with activity against Mtb , but we extend these results here to Stm as well. These data again show the validity of our screening and prediction approach since we are able to consistently and faithfully confirm already-available knowledge. The data on haloperidol also suggest that this compound may be applicable for HDT in a broader spectrum of intracellular bacterial infections. The second hit compound, mibefradil, is a Ca 2+ channel blocker [61] . The majority of screening hits in the HeLa- Stm infection model exacerbated bacterial loads and even though these compounds can therefore not be used for drug repurposing, all of the identified compounds may be important starting points for gaining deeper mechanistic insight into Stm –host interactions. The limited overlap between the hit compounds from Mtb and Stm screens likely reflects the vastly different intracellular “lifestyles” of these pathogens. Notwithstanding this, several compounds display consistent intracellular antimicrobial activity in both Mtb and Stm infection models, such as haloperidol. These compounds are therefore promising candidate drugs with wider application against (antibiotic resistant) intracellular bacterial infections. Selecting hits for follow-up analysis in large (chemical) screens poses substantial challenges. Here, we employed two complementary strategies for screening follow-up. First, as we aimed to identify compounds with superior host-directed antimicrobial activity, we focused on compounds performing better than the reference compound H-89, resulting in a strictly data-driven hit cutoff. Using this strategy, we identified SU 6656, quinacrine, SB 216763, GW5074, and tyrphostin AG 494 as the most promising candidate compounds for TB and mibefradil for salmonellosis, as well as confirmed haloperidol as an attractive drug for HDT against both Mtb and Stm . Second, as screening outcome may be strongly influenced by compound properties such as solubility, hydrophobicity, concentration, IC 50 , and target selectivity, using a strict cutoff may mask valuable data hidden in the large data set and will be lost to follow-up. We therefore used a complementary follow-up approach by developing an innovative in silico compound predictive model to uncover relevant chemical compound classes and target profiles in screening data. Focusing on confirmed target profiles by automated extraction of bioassay data from PubChem, we were able to both discern compound targets and predict novel active compounds. As the target profiles were ranked without using a hit cutoff, this approach enabled unbiased validation and follow-up of the primary chemical compound screen. The use of simple numerical values as predictive parameters renders this prediction model highly adaptable and easily applicable to other chemical screens. The model significantly enhanced the identification of de novo hit compounds (55.6% and 50% for Mtb and Stm , respectively) compared to random LOPAC library primary screening (10% for Mtb and 14.6% for Stm ). Remarkably, the predicted Mtb hit compounds AT9283, ENMD-2076, and dovitinib were all (growth factor) RTK inhibitors [47] , [48] , [49] . As inhibitors of RTK signaling molecules were already observed to be overrepresented in the hits from our drug-repurposing screen, our predictive model successfully provided an unbiased validation of this observation and prompted us to further focus our screening endeavor on RTK inhibitors. RTK inhibitors are widely studied in cancer research for their antineoplastic properties [62] . Phase II clinical trials have been performed with both AT9283 and ENMD-2076 and dovitinib has already passed phase III clinical trials [63] , [64] , [65] , [66] , [67] , [68] ( http://www.clinicaltrials.gov ), enabling swift future drug repurposing as host-directed antimicrobials. Our unbiased siRNA screen of the human kinome independently identified and validated RTK signaling as a host pathway regulating Mtb survival, identifying BLK, ABL1, and NTRK1 as host kinases, and controlling intracellular Mtb and possible drugable targets. BLK is an SFK involved in B cell receptor signaling and the insulin response to glucose uptake in pancreatic islet cells [69] , [70] . The non-receptor tyrosine kinase ABL1 was previously linked to mycobacterial infection and its commonly used inhibitor imatinib was shown to exert host-directed Mtb-inhibiting activity in vivo [15] , [21] , providing independent validation of our siRNA screening. Finally, NTRK1 is an RTK involved in peripheral nervous system development and synaptic function and plasticity [71] . Various cells of the hematopoietic lineage have been shown to produce the NTRK ligand nerve growth factor during inflammation and autoimmunity [72] and expression of NTRKs in monocytes has been previously reported [73] . Next to the confirmation of these compound targets by genetic silencing as described here, there were other siRNA hits involved in RTK signaling which might represent as-yet-unknown molecular targets for these or other hit compounds. Conversely, confirmed compound targets that were not identified in our siRNA screen may still contribute to Mtb control due to redundancy and possible incomplete genetic knockdown inherent to siRNA screens. A role for growth factors in mycobacterial infection has been previously reported. The growth factor VEGF was linked to mycobacterial infection in a zebrafish Mycobacterium marinum ( Mmar ) infection study [28] as well as in a rabbit Mtb infection model [27] . However, in both studies, the reported effect of VEGF was primarily systemic rather than (sub)cellular, inducing enhanced angiogenesis in granulomas. Our data strongly suggest that an intracellular response to growth factor receptor signaling via RTKs may be another important determinant for mycobacterial infection outcome. Interestingly, Oehlers et al. used pazopanib, one of the compounds identified by our predictive model to show an inhibitory effect of VEGF receptor (VEGFR) inhibition on vascularization around nascent granulomas in their model. Though not meeting our strict hit selection criteria, pazopanib statistically significantly ( z -score –1.50) decreased Mtb loads in our screen (and thus in the absence of a vascular system), suggesting that cellular Mtb inhibition by pazopanib might precede or complement the vascularization effects observed in vivo by Oehlers et al. Additionally, epidermal growth factor receptor (EGFR) signaling has previously been linked to mycobacterial infection through a chemical screen identifying EGFR inhibitor gefitinib as a compound that restricts Mtb growth [31] . Our study significantly expands this knowledge by introducing additional RTK-targeting compounds that can be used for drug repurposing, including compounds targeting VEGFR (dovitinib) and EGFR (tyrphostin AG 494) signaling. Our in silico predictive model successfully identified two compounds (nafoxidine, an estrogen receptor modulator and opipramol, a sigma receptor agonist) with host-directed Stm -inhibiting activity. Interestingly, haloperidol (a hit in both the Mtb and Stm LOPAC screens) was previously reported to interact with sigma receptors with high affinity [74] , suggesting mechanistic involvement of sigma receptors in host control of intracellular bacteria. Finally, the development and validation of a novel fluorescence-based screening assay that is able to rapidly quantify intracellular bacterial infection in human cells, as described here, we think that it is important since it helps shortening the readout from a classical 3-week CFU assay for Mtb to 24–72 h using flow cytometry. The assay is highly reproducible, medium throughput, provides an excellent assay window, and is suitable for screening both chemical compound and siRNA libraries. Taking advantage of the previously reported phagocytic capability of melanocytes [41] , we also report the human melanoma cell line MelJuSo as a novel model for Mtb infection studies, particularly for studies encompassing chemical and RNAi screens. Importantly, our assay faithfully reproduces the inhibitory effect of several previously published host-directed compounds (that were identified using different strategies, approaches, and models) on Mtb intracellular survival, as well as HDT results obtained in human primary macrophages, further validating our novel infection model. In conclusion, the results from our chemical, genetic, and novel bioinformatics approach provide an important proof of concept of HDT for intracellular infections, such as (MDR) TB and salmonellosis. Moreover, our results identify human RTK signaling as a signaling pathway targetable by novel repurposable drugs, providing a new and promising therapeutic starting point for drug development against Mtb , including MDR- Mtb . Reagents H-89 dihydrochloride, D4476, IC261, LY-364947, DAPH 2, nafoxidine hydrochloride, 1,3-di-o-tolylguanidine, naftifine hydrochloride, opipramol, rifampicin, kanamycin, and the library of pharmacologically active compounds (LOPAC) were purchased from Sigma-Aldrich, Zwijndrecht, the Netherlands. Hygromycin B was acquired from Life Technologies-Invitrogen, Bleiswijk, the Netherlands. Imatinib mesylate was from Enzo Life Sciences, Raamsdonksveer, the Netherlands. VEGFR2 kinase inhibitor I and ampicillin were purchased from Calbiochem Merck-Millipore, Darmstadt, Germany. Pazopanib HCl, AT9283, and linifanib (ABT-869) were acquired from Selleck Chemicals, Munich, Germany. Quizartinib was purchased from MedChemExpress, Stockholm, Sweden. Santa Cruz BioTechnology, Heidelberg, Germany was the supplier of PDGFR tyrosine kinase inhibitor III. Dovitinib (TKI-258, CHIR-258) was from APExBIO, Houston, TX, USA. The siKinome library was acquired from Thermo Fisher Dharmacon, Waltham, MA, USA. Cell culture HeLa cells and the MelJuSo human melanoma cell line were maintained at 37 °C and 5% CO 2 in Gibco Iscove’s Modified Dulbecco’s Medium (IMDM; Life Technologies-Invitrogen) with 10% fetal bovine serum (FBS, Greiner Bio-One, Alphen a/d Rijn, the Netherlands), 100 units/ml penicillin and 100 µg/ml streptomycin (Life Technologies-Invitrogen). Proinflammatory Mφ1s and anti-inflammatory Mφ2s were generated from monocytes isolated from whole blood of healthy donors by FICOLL separation and CD14 MACS sorting (Miltenyi Biotec, Teterow, Germany) followed by 6 days of differentiation with 5 ng/ml granulocyte macrophage–colony-stimulating factor (GM–CSF; BioSource Life Technologies-Invitrogen) or 50 ng/ml macrophage–colony-stimulating factor (M–CSF; R&D Systems, Abingdon, UK), respectively, as previously reported [75] . Mφs were cultured in Gibco Roswell Park Memorial Institute (RPMI) 1640 medium (Life Technologies-Invitrogen) with 10% FBS and 2 mM L-alanyl-L-glutamine (PAA, Linz, Austria). Bacterial culture Bacterial strains used are displayed in Supplementary Table 1 . Mycobacteria were cultured in Difco Middlebrook 7H9 broth (Becton Dickinson, Breda, the Netherlands) supplemented with 10% ADC (Becton Dickinson), 0.5% Tween-80 (Sigma-Aldrich), and appropriate antibiotics. Stm was cultured on Difco Luria-Bertani (LB) agar (Becton Dickinson) or in Difco LB broth (Becton Dickinson) supplemented with appropriate antibiotics. Stm and Mtb infections One day before infection, mycobacterial cultures were diluted to a density corresponding with early log-phase growth (optical density at 600 nm (OD 600 ) of 0.4). Stm was grown either in LB broth or on LB agar with appropriate antibiotics. After overnight incubation, Stm liquid cultures were diluted 1:33 and cultured for an additional 3–4 h, while plate-grown Stm was suspended in PBS by rinsing the agar plates. Bacterial density was determined by measuring the OD 600 and the bacterial suspension was diluted in cell culture medium without antibiotics to reach a multiplicity of infection (MOI) of 10 (unless indicated otherwise). Accuracy of bacterial density measurements was verified by a standard colony-forming unit (CFU) assay. Cell cultures (HeLa for Stm infections and MelJuSo for Mtb infections), seeded in 96-well flat-bottom plates as described below, were inoculated with 100 μl of the bacterial suspension, centrifuged for 3 min at 800 rpm, and incubated at 37 °C/5% CO 2 for 20 min if infected with Stm or 60 min if infected with Mtb . The plates were then washed with culture medium containing 30 μg/ml gentamicin sulfate (Lonza BioWhittaker, Basel, Switzerland) and incubated at 37 °C and 5% CO 2 in a medium containing 5 μg/ml gentamicin and the indicated chemical compounds until readout by flow cytometry or CFU, as indicated. Chemical compound treatment A total of 10,000 HeLa or MelJuSo cells were seeded per well in 96-well flat-bottom plates or 300,000 primary macrophages were seeded per well in 24-well plates in appropriate culture medium without antibiotics 1 day prior to infection with Mtb or broth-grown Stm . Infected cells were treated overnight with chemical compounds at 10 μM (unless indicated otherwise) or DMSO at equal v/v in a medium containing 5 μg/ml gentamicin. siRNA transfections A total of 3,000 HeLa or MelJuSo cells were reverse-transfected with ON-TARGETplus siRNA pools (Thermo Fisher Dharmacon, Waltham, MA, USA) at a 50 nM concentration using 0.2 μl of Dharmafect1 (Thermo Fisher Dharmacon) per well in a flat-bottom 96-well plate in appropriate culture medium without antibiotics. Knockdown efficiency was verified by immunoblotting at the indicated time points. Cells transfected with siRNA were infected with Mtb at MOI 1000 24 h post transfection and incubated for an additional 48 h and infections with agar-grown Stm were carried out at MOI 500 72 h post transfection and incubated overnight, unless indicated otherwise. Colony-forming unit assay CFU assays were performed using the track dilution method described previously [76] . In short, bacterial suspensions were serially diluted and 10-μl drops were plated on square agar plates, which were subsequently placed at an angle to allow the drops to spread over a larger surface area. Bacterial growth assay A volume of 100 μl of Stm or Mtb culture (OD 600 of 0.1) was plated in a flat-bottom 96-well plate containing 100 μl of indicated chemical compounds at 20 μM in LB ( Stm ) or 7H9 ( Mtb ) broth. The plate was incubated at 37 °C overnight for Stm or during a period of 15 days for Mtb and absorbance was measured at a 550-nm wavelength on a Mithras LB 940 plate reader (Berthold Technologies, Bad Wildbad, Germany). Fluorescence microscopy A total of 100,000 HeLa or MelJuSo cells were grown on glass coverslips (Menzel-Gläser, Braunschweig, Germany) in 24-well plates and infected as described above. Samples were fixed for 30 min at RT with 4% paraformaldehyde, embedded in VectaShield with DAPI (Brunschwig Chemie, Amsterdam, the Netherlands), and examined on an Axioskop 2 fluorescence microscope (Carl Zeiss, Sliedrecht, the Netherlands). STRING analysis Protein interaction networks were generated using STRING version 10 ( http://string-db.org/ ) [77] using experiments and databases as data sources and a minimal confidence score of 0.4. Statistics Student’s t test, one-way ANOVA, and linear regression were performed using GraphPad Prism version 6.0 for Mac OS X (GraphPad Software, San Diego, CA, USA; www.graphpad.com ). Data availability The data that support the findings of this study are available from the corresponding authors on request. Code availability The code of the machine-learning software CLUS that was used to build the in silico models for predicting compound activity is available for download from the SourceForge repository (at https://sourceforge.net/projects/clus/ ).